Meta-analysis of gene–environment-wide association scans accounting for education level identifies additional loci for refractive error Myopia is the most common human eye disorder and it results from complex genetic and environmental causes. The rapidly increasing prevalence of myopia poses a major public health challenge. Here, the CREAM consortium performs a joint meta-analysis to test single-nucleotide polymorphism (SNP) main effects and SNP × education interaction effects on refractive error in 40,036 adults from 25 studies of European ancestry and 10,315 adults from 9 studies of Asian ancestry. In European ancestry individuals, we identify six novel loci ( FAM150B-ACP1 , LINC00340 , FBN1 , DIS3L-MAP2K1 , ARID2-SNAT1 and SLC14A2 ) associated with refractive error. In Asian populations, three genome-wide significant loci AREG , GABRR1 and PDE10A also exhibit strong interactions with education ( P <8.5 × 10 −5 ), whereas the interactions are less evident in Europeans. The discovery of these loci represents an important advance in understanding how gene and environment interactions contribute to the heterogeneity of myopia. Myopia, or nearsightedness, has rapidly emerged as a global health concern in the last three decades [1] . It is one of the leading causes of visual impairment and is associated with potentially blinding ocular complications including myopic maculopathy, glaucoma, cataract and retinal detachment [2] . Evidence from family and twin studies strongly supports the heritability of myopia [3] . Estimates for the heritability of the quantitative trait refractive error have been reported to be as high as 90% (ref. 4 ). On the other hand, the rapid upsurge of myopia in the last few decades in many parts of the world is likely to be a consequence of lifestyle changes such as the increasing educational intensity, in particular in urban East Asia [5] , [6] , and potentially gene and environment (G × E) interactions. Major attempts undertaken in genome-wide association studies (GWAS) to elucidate the genetic determination of myopia and refractive error have recently led to the discovery of >30 distinct susceptibility loci [7] , [8] . Nevertheless, collectively these genetic variants are estimated to explain <12% of phenotypic variance in refractive errror [7] , [8] . As myopia is a result of the combination of genetic and environmental factors, interplay between genes and environment may account for a substantial proportion of the phenotypic variance. In recent times, we showed interactions between education and genetic risk score of myopia derived from 26 known GWAS single-nucleotide polymorphisms (SNPs) in the Rotterdam Study [9] ; the combined effect of genetic predisposition and education on the risk of myopia was substantially greater than anticipated from a simple sum of these two factors. At the gene level, some genes such as SHISA6-DNAH9 have been shown to interact with education level and exhibit strong genetic effects for myopia among Asians with at least higher secondary education [10] . In the current study, we demonstrate that new genetic effects implicated in myopia development could be uncovered by studying interactions between genetic variants and education level. In the context of the aetiology of refractive errors, education attainment is generally considered a surrogate measure for accumulated near work activity [1] . When viewing near objects, the eye generates extra optical power through the process of accommodation to focus the image on the retinal plane, to maintain clear vision [11] . There is an accommodative lag (less accommodation produced than needed) in many myopes, resulting in a hyperopic defocus on the retina for near work, which has long been proposed to promote eye growth [1] , [12] , but whether this occurs before or after the onset of myopia in humans is less clear. The retina has a central role in the mechanism linking such visual input with eye growth and refractive development [13] . Several neurotransmitters or molecules have been implicated in this process by animal studies including dopamine, acetylcholine, vasoactive intestinal peptide, GABA (γ-aminobutyric acid) and glucagon [14] , [15] . However, an organized framework for the retinal signalling mechanisms underlying refractive error development under various environmental conditions remains to be elucidated. Factoring in environmental exposures may enhance power for the detection of genes, especially in circumstances where a genetic locus has a differential effect conditional on specific environment exposures [16] . Gene–environment-wide interaction studies (GEWIS) using a joint meta-analysis (JMA) approach on SNP main effects and SNP × environment interactions have recently been described [17] , [18] . This approach has successfully identified six novel loci associated with fasting insulin and glucose accounting for interactions with body mass index [18] . It also led to the identification of two novel loci for pulmonary function that did not emerge from analyses based on the genetic main effects alone [19] . The well-documented effects of educational attainment on myopia and refractive error make the proposed interaction an excellent analytical candidate for the GEWIS. The availability of large-scale GWAS spherical equivalent data sets from the Consortium for Refractive Error And Myopia (CREAM) makes G × E interaction analyses feasible. To identify additional genetic variants for refractive error, we performed GEWIS-based analyses on 40,036 adults of European ancestry from 25 studies and 10,315 adults of Asian ancestry from 9 studies. We identified nine new loci using the JMA approach, where three loci exhibited G × E interaction on refractive error in Asians, including the GABA C receptor subunit ρ1 gene GABRR1 . 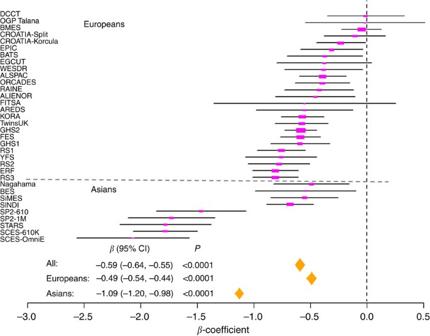Figure 1: Forest plot of education main effects on spherical equivalent across studies. Theβ-coefficient represents the differences of dioptres in refractive error comparing individuals in higher education group versus lower education group in Europeans (n=40,036), Asians (n=10,315) and all studies (n=50,351). The studies are sorted by effect size of education on spherical equivalent within Europeans and Asians studies, respectively. Educational level and its main effects on spherical equivalent The baseline characteristics of 50,351 participants from 34 studies in our meta-analysis are shown in Table 1 . A total of 40,036 participants were of European descent and 10,315 were of Asian descent; the age of the participants ranged from 20 to 99 years. We grouped individuals into two educational categories: a higher education group that included individuals who completed higher secondary or university education and a lower education group comprising those with lower secondary education or below (see Methods). Among Europeans, the proportions of participants in the higher education group ranged from 16.5% (FITSA [20] and OGP Talana [21] ) to 94.4% (AREDS [22] ) with an average of 50.7% ( Supplementary Table 1 ). In Asians, the proportions of individuals in the higher education group ranged from 6.7% (SiMES [23] ) to 75.9% (Nagahama [24] ) with an average of 30.0%. Across all studies, individuals in the higher education group had a spherical equivalent refractive error that was on average 0.59 dioptres (D) more myopic, or less hyperopic, compared with those in the lower education group ( β =−0.59 D; 95% confidence interval (CI): −0.64 to −0.55 D). High education level was associated with a twofold more myopic spherical equivalent in individuals of Asian as compared with European ancestry (Asians: β =−1.09 D, 95% CI: −1.20 to −0.98 D; Europeans: β =−0.49 D, 95% CI: −0.54 to −0.44 D; Fig. 1 ). Among Asian studies, we also observed heterogeneity of education effects for refractive error. The education effects on spherical equivalent in Singapore Chinese were significantly larger than that in other Asian studies (Singapore Chinese: β =−1.75 D, 95% CI: −1.92 to −1.58 D; other Asian cohorts: β =−0.60 D, 95% CI: −0.75 to −0.46 D). Table 1 Characteristics of study participants. Full size table Figure 1: Forest plot of education main effects on spherical equivalent across studies. The β -coefficient represents the differences of dioptres in refractive error comparing individuals in higher education group versus lower education group in Europeans ( n =40,036), Asians ( n =10,315) and all studies ( n =50,351). The studies are sorted by effect size of education on spherical equivalent within Europeans and Asians studies, respectively. 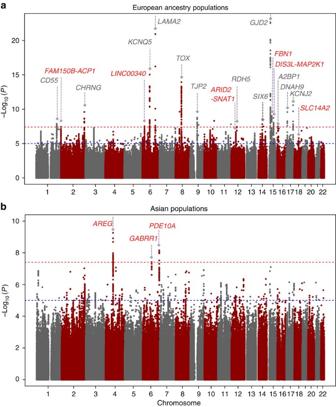Figure 2: Manhattan plots of −log10(P) for the JMA on SNP main effects and SNP × education effects on spherical equivalent in (a) European ancestry populations and (b) Asian populations. The horizontal red line indicates the genome-wide significance level ofPJMA<5 × 10−8. The horizontal blue line indicates the suggestive significance level ofPJMA<1 × 10−5. Novel loci reaching genome-wide significance are labelled in red and known loci are in grey. Full size image GEWIS in Europeans After stringent quality control (QC) filtering, ∼ 6 million SNPs in each study were eligible for the genome-wide JMA test ( Supplementary Table 2 ). The JMA for SNP main effects and SNP × education interactions in 40,036 European Ancestry individuals showed an association with spherical equivalent at 12 previously implicated loci ( Fig. 2a , Supplementary Table 3 and Supplementary Fig 1 ). We also identified four previously unreported loci associated with spherical equivalent achieving genome-wide significance ( P JMA <5.0 × 10 −8 ; P het ≥0.086; Table 2 ): FAM150B-ACP1 , LINC00340 , FBN1 and DIS3L-MAP2K1 . The significant association for JMA testing at these loci in Europeans was primarily driven by SNP effects in both the lower and higher education strata (4.40 × 10 −8 ≤ P main ≤1.35 × 10 −6 and 7.61 × 10 −11 ≤ P main ≤1.75 × 10 −6 , respectively). SNP × education interaction was not significant ( P int ≥0.208). The estimated effect sizes of SNP effects on spherical equivalent were highly similar across education strata. Figure 2: Manhattan plots of −log 10 ( P ) for the JMA on SNP main effects and SNP × education effects on spherical equivalent in (a) European ancestry populations and (b) Asian populations. The horizontal red line indicates the genome-wide significance level of P JMA <5 × 10 −8 . The horizontal blue line indicates the suggestive significance level of P JMA <1 × 10 −5 . Novel loci reaching genome-wide significance are labelled in red and known loci are in grey. Full size image Table 2 Six genetic loci associated with spherical equivalent from the JMA in the European populations and combined analyses. Full size table GEWIS in Asians The JMA for spherical equivalent in 10,315 individuals from the Asians cohorts identified genome-wide significant association for three genes: AREG , GABRR1 and PDE10A ( P JMA <5.0 × 10 −8 ; Table 3 and Fig. 2b ). SNP × education interaction effects associated with spherical equivalent were observed at all three loci, with genetic effects significantly larger within participants who had a higher level of education compared with those with a lower education level: AREG (rs12511037, β int =−0.89±0.14 D, P int =6.87 × 10 −11 ), GABRR1 (rs13215566, β int =−0.56±0.14 D, P int =8.48 × 10 −5 ) and PDE10A (rs12206610, β int =−0.72±0.13 D, P int =2.32 × 10 −8 ). The genotype and phenotype associations were highly significant in the higher education stratum (main genetic effects, 1.97 × 10 −10 ≤ P main ≤8.16 × 10 −8 ) but were considerably weaker in the lower education stratum (0.008≤ P main ≤0.243). There was no evidence of inter-study heterogeneity at index SNPs within AREG , GABRR1 or PDE10A loci ( Q -test: P het ≥0.122). Table 3 Three genetic loci associated with spherical equivalent with a significant SNP × education interaction in Asians and results in European populations. Full size table GABRR1 and PDE10A index SNPs were not associated with spherical equivalent in European samples, for either the JMA test, SNP main effect or SNP × education interaction ( Table 3 ). AREG SNP rs12511037 was excluded in the meta-analysis of European studies after QC filtering; hence, a proxy SNP, rs1246413, in linkage disequilibrium (LD) with rs12511037 in Asians ( r 2 =0.97) was tested but not associated with spherical equivalent ( P JMA =0.527; P int =0.176). The meta-regression including study-level characteristics as covariates in the model confirmed the heterogeneity between populations of European and Asian ancestry ( GABRR1 : P =0.006; PDE10A : P =0.0419; Supplementary Table 4 ). For PDE10A , besides ethnicity, average spherical equivalent of each study also explained the inter-study heterogeneity for the interaction effects ( P =0.025). We examined whether the underlying assumption of G × E independence held at these three G × E interaction loci. We performed a meta-analysis of logistic regression analysis for education level on AREG SNP rs12511037, GABRR1 SNP rs13215566 and PDE10A SNP rs12296610, adjusting for age, gender and population stratification in Asian cohorts ( n =10,315). Our analysis did not reveal any significant associations between these loci and education level ( P ≥0.102, P het ≥0.170; Supplementary Table 5 ). Furthermore, the three loci were not associated with educational attainment in a large meta-analysis of GWAS recently conducted in European cohorts [25] . Thus, our G × E results are unlikely to be biased due to dependence between gene and education. We also evaluated the association for spherical equivalent in Asian cohorts for four loci identified from European populations. Two of them showed significant associations in the JMA test: FAM150B-ACP1 ( P JMA =0.031) and DIS3L-MAP2K1 ( P JMA =0.0042; Table 2 ). The SNP effect sizes in lower and higher education strata in Asians were similar at FAM150B-ACP1 . The signal at the DIS3L-MAP2K1 locus was mainly driven by SNP × education interaction in Asians ( P int =7.95 × 10 −4 ), whereas the interaction effect was not statistically significant in Europeans ( P int =0.208). Combined GEWIS of all cohorts We subsequently conducted a JMA in the combined data including both the European and Asian participants of all 34 studies. This analysis revealed two additional SNPs: ARID2-SNAT1 ( P JMA =4.38 × 10 −8 ) and SLC14A2 ( P JMA =2.54 × 10 −8 ). Both loci showed suggestive association with spherical equivalent in European cohorts, with the same direction of effect and similar effect sizes in Asian cohorts ( Table 2 ). We also detected genome-wide significant associations with spherical equivalent for 17 known loci [8] identified in our previous CREAM GWAS ( Supplementary Table 3 ). The regional plots of the identified novel loci are presented in Supplementary Fig 2 . Gene and education interactions for GWAS known loci We also evaluated the interactions between education and previously reported genetic association with spherical equivalent at 39 loci identified from recent two large GWAS studies [7] , [8] . Two SNP × education interactions were nominally significant ( Supplementary Table 6 ): TJP2 in Europeans (rs11145488, P int =6.91 × 10 −3 ) and SHISA6-DNAH9 in Asians (rs2969180, P int =4.02 × 10 −3 ). In general, the index SNPs tested at 39 loci had larger SNP × education interaction effect on spherical equivalent in Asians versus Europeans (meta-regression P for fold changes<0.001; Supplementary Fig. 3 ). For 20 SNPs with the same direction of the interaction effect, the magnitudes of interaction effects were fourfold larger on average in Asians than in Europeans ( P =0.003). Gene and near work interactions for three identified loci High education levels may reflect an estimator for the greater accumulative effect of near work [26] , [27] . We thus examined whether there was evidence for SNP × near work interactions associated with spherical equivalent at the three loci ( AREG , GABRR1 and PDE10A ) in paediatric cohorts (SCORM [28] , Guangzhou Twins [29] and ALSPAC [30] ; combined n =5,835; Supplementary Table 7 ). Tentative support for a SNP × near work interaction was observed for PDE10A (rs12206610, P int =0.032, P het =0.658), with the stronger genetic effect in children spending more hours on reading, writing or compute use. Weaker support for an interaction was noted at GABRR1 (rs13215566, P int =0.309, P het =0.655), although the direction of meta-analysed interaction effect was largely consistent across paediatric studies with that observed in adults. We did not observe the interaction at AREG (rs12511037, P int =0.795, P het =0.062). Gene expression in human tissues Using the Ocular Tissue Database [31] , we examined the expression of the associated genes in 20 normal human donor eyes. The majority of genes identified were expressed in human retina, sclera, choroid or retinal pigment epithelium (RPE) ( Supplementary Table 8 ). Among these genes, GABRR1 , ACP1 and SNAT1 had the highest expression in the retina. The Probe Logarithmic Intensity Error-normalized messenger RNA expression levels in the retina ranged from 121.66 to 236.69. Of note, MAP2K1 was widely expressed in the retina, sclera and choroid/RPE. This study represents the most comprehensive genome-wide scan of gene and education interactions to date, for refractive error. Here we identified novel genetic loci associated with refractive error by testing the joint contribution of SNP main effects and SNP × education effects in large multi-ethnic populations. Three loci ( AREG , GABRR1 and PDE10A ) showed strong interactions with education in populations of Asian descent, with larger genetic effects within participants who had a higher level of education compared with those with a lower education level; no interactions achieved statistical significance in Europeans for top JMA associations or known myopic loci. Apart from confirming known associations at 17 previous published loci, we identified six new loci ( FAM150B-ACP1 , LINC00340 , FBN1 , DIS3L-MAP2K1 , ARID2-SNAT1 and SLC14A2 ) significantly associated with spherical equivalent using the combined multi-racial cohort. A recent meta-analysis of GWAS in multi-ethnic populations comprises 32 studies ( n =45,756) from CREAM and a large GWAS in Europeans ( n =45,771) have reported a total of 39 genetic loci associated with refractive phenotypes [7] , [8] . The current genome-wide meta-analysis included ∼ 5,000 more subjects than the previous GWAS of main effects. We identified nine additional novel loci using the JMA approach. These loci can be placed within the biological context of the visually evoked signalling cascade that begins in the retina and mediates sclera remodelling [32] . The newly identified genes are involved in retinal neurotransmission ( GABRR1 and SNAT1 ), extracellular matrix remodelling ( FBN1 , MAP2K1 and AREG ), circadian rhythm ( PDE10A ) and platelet-derived growth factor receptor signalling ( ACP1 ) ( Supplementary Table 9 ). Network analysis revealed that most of the novel genes may tend to be co-expressed and co-localized with the known myopia susceptibility genes through multiple biological networks such as LAMA2 , GJD2 , RASGRF1 , BMP3 , RDH5 , ZMAT4 , RBFOX1 , RDH5 and so on ( Supplementary Fig. 4 ). Our data, in line with previous findings, substantiate the assumption of heterogeneity in the molecular mechanisms involved in refractive error and myopia. Among the novel loci, GABRR1 on chromosome 6q15 (53 kb), encoding GABA C receptor subunit ρ1, is an interesting functional candidate suggestive of a role in myopia development. Modulation of synaptic plasticity via GABA-mediated inhibition would be well placed to alter the ‘gain’ of the visually guided feedback system controlling refractive development [33] . The lead SNP rs13215566 in GABRR1 , together with seven SNPs within the LD block ( r 2 ≥0.8), are intronic, potentially affecting regulatory motifs (such as zfp128 and gcm1) that may influence transcriptional regulation ( Supplementary Table 10 ). The variant rs13215029, in LD ( r 2 =1) with rs13215566, is associated with cis -acting expression of GABRR1 ( P =2.3 × 10 −4 ) in skin tissues ( Supplementary Table 9 ) [34] . A recent pharmacological study provided evidence that retinal dopaminergic and GABAergic neurotransmitters play a substantial role in the modulation of refractive development in form-deprivation myopia [35] , [36] , [37] . Stone et al . [35] have reported that antagonists to GABA-A, -B and -C receptors inhibited form-deprivation myopia in chicks, with greatest effect in the equatorial dimension. GABA receptors, expressed in bipolar and ganglion neuron cells, also interact with dopamine pathways in the retina [36] . A recent proteomics study determined that levels of GABA transporter-1 were significantly reduced in myopic murine retina after atropine treatment, implying that GABA signalling is involved in the anti-myopic effects of atropine [37] . Altogether, these data suggest that GABA C receptor ρ1 may regulate the development of myopia through functional feedback from RPE to neuron cells in the retina. Further studies are needed to investigate the effect of genetic deletion of GABRR1 on refractive eye development and the role of the GABAergic pathway in myopia development using gene knockout mice. Therefore, our result in humans is in line with animal experiments, supporting the notion that the GABAergic neurotransmitter signalling pathway in the retina could be a potential factor in the progression of myopia. SNP rs10889855 on chromosome 6 is an intronic variant within the ARID2 gene (AT-rich interactive domain 2) and 500 kb downstream of SNAT1 (solute carrier family 38, member, alias SLC38A1 ). SNAT1 is a transporter of glutamine, a precursor of GABA [38] . It is also highly expressed in human retina. In our previous meta-analysis in CREAM [8] , we identified variants in another glutamate receptor gene GRIA4 (encoding glutamate receptor, ionotropic); altogether, current evidence supports the notion that retinal neurotransmitters GABA and glutamine may be involved in the refractive development. The strongest association signal for gene and environment interactions was from rs12511037, located 14 kb downstream the AREG gene (amphiregulin). AREG is a ligand of the epidermal growth factor receptor promoting the growth of normal epithelial cells, which is critical for cell differentiation and proliferation such as regrowth of the wounded cornea [39] . A link has been found between the muscarinic acetylcholine receptors, dominant in myopia progression, and the epidermal growth factor receptor in muscarinic system [40] , [41] . Another novel association, rs16949788 on chromosome 15, derives from a region that spans DIS3L and MAP2K1 . MAP2K1 encodes mitogen-activated protein kinase 1, which binds to muscarinic receptors during proliferation [42] and inhibits the proliferation of human scleral fibroblasts exposed to all- trans retinoic acid [43] . All- trans retinoic acid is a modulator of ocular growth, inhibiting the proliferation of human scleral fibroblasts [44] . FBN1 (Fibrillin 1), a member of the fibrillin family, encodes a large extracellular matrix glycoprotein. Mutations in FBN1 cause Marfan’s syndrome, a disorder of connective tissue affecting the ocular, skeletal and cardiovascular systems [45] . As a candidate gene for myopia, attempts to study its association with myopia previously produced inconclusive results [46] , [47] , probably owing, in part, to underpowered studies with insufficient sample sizes. Using data from a large multi-ethnic population, our results support the role of FBN1 in myopia development. The genome-wide significant SNPs from the JMA approach did not exhibit any interactions with education in Europeans, in contrast to the significant interactive effect among Asians. In particular, the G × E interactions at AREG , GABRR1 and PDE10A were only evident in Asian populations. There are a number of possible reasons for the observed differences. First, the variation of LD patterns and joint effects of genetic variants might affect the transferability of G × E signals across populations. Similar LD patterns were seen at GABRR1 and PDE10A regions across populations whereas a long stretch of LD flanking AREG was present only in Asian populations ( Supplementary Fig. 5 ). As the true causal variants transferrable across populations are probably not implicated in our study, the identified novel myopia risk loci provide a much-needed starting point for follow-up and functional downstream analyses. Second, we used education level in adults as a surrogate measure of the underlying risk factors for influencing refractive development. Ideally, near work intensity would be measured prospectively in children before the onset of myopia. Studies included in our analyses do not have additional data on relevant childhood exposures. Thus, the best available surrogate measure of cumulative near work exposure in adult cohorts is educational level. We nevertheless believe that education is a highly reliable proxy for the relevant exposures underlying refractive development and is universally associated with refractive error in our study. Third, the differences of G × E interactions in Asian versus Europeans may reflect quantitative differences in near work intensity during childhood. For example, 6- and 7- year-old children in England and Australia reported less near work activity outside of school (1.0–2.3 h per day) [48] , [49] compared with children in Singapore and China (2.7–3.5 h per day) [50] , [51] . A similar trend was observed in older children [48] , [52] , [53] , [54] , [55] . We thus speculate that the total exposure to near work activity may be greater in East Asians compared with European-derived populations with the same levels of education; hence, G × E interaction estimates would tend to be inflated in Asian populations compared with European groups. Fourth, other environmental factors such as outdoor activities could also interact with genes. East Asian children tend to have less exposure to outdoor activities compared with their European peers [56] . However, the majority of adult cohorts did not report time outdoors and thus could not be accounted for in the current study. Finally, the population mean of refractive error is less myopic in Europeans (0.10 D) versus Asians (−0.60 D). Of note, for the previously known myopia loci, the magnitudes of interaction effects were fourfold larger on average in Asians than in Europeans ( Supplementary Fig. 2 ). The impact of G × E interactions may be seen at certain severity levels of myopia. The risk alleles of rs12511037 in AREG , rs1321556 in GABRR1 and rs12206610 in PDE10A had no or weak influence on myopic shift in the lower education group compared with the higher education group. This suggests that the hereditary predisposition to myopia could be latent for the risk allele carriers, if they are less exposed to the myopiagenic environment associated with high-level education. A lack of strong SNP × near work associations in children might be due to the inadequate statistical power in paediatric cohorts of relatively small sample sizes, or the possibility that environmental risk exposures other than near work might underlie the SNP × education interaction seen in the adult Asian samples. In summary, we identified nine novel loci associated with refractive error in a large multi-ethnic cohort study by GEWIS approach. Our data provide evidence that specific genetic variants interact with education, to influence refractive development, and further support a role for GABA neurotransmitter signalling in myopia development. These findings provide promising candidate genes for follow-up work and may lead to new genetic targets for therapeutic interventions on myopia. Study participants Thirty-four studies from members of CREAM, comprising 40,036 individuals of European ancestry from 25 studies and 10,315 individuals of Asian ancestry from 9 studies, were made available for this analysis ( Table 1 and Supplementary Note 1 ). Individuals aged <20 years were excluded and so were those who had undergone cataract surgery, laser or other intra-ocular procedures that could alter refraction. Many of these studies were also included in the previous CREAM GWAS on spherical equivalent [8] . All studies adhered to the tenets of the Declaration of Helsinki and were approved by their local research ethics committees. The exact names of the Institutional Research Board committees can be found under Supplementary Note 2 . All participants provided a signed consent form before the start of the study. Phenotyping and education levels All participants underwent ophthalmological examinations ( Supplementary Table 1 ). Non-cycloplegic refraction was measured by autorefraction and/or subjective refraction. Spherical equivalent was calculated as the sphere power plus half of the cylinder power for each eye. The mean spherical equivalent of the right and left eyes was used as a quantitative outcome. When data from only one eye was available, the spherical equivalent of that eye was used. For each study, the participants reported the highest level of education achieved or the years of schooling through a self-reported questionnaire, or in an interview. We dichotomized education for all participants in each study. The higher education group consisted of those who had achieved the highest educational level of A-levels, high school (higher secondary education), vocational training (for example, diploma), university degree or those with ≥12 years spent in formal education (beginning from first grade). Those who had achieved the highest educational level of O-level, middle school (lower secondary education) or those with <12 years of formal education were classified into the lower education group. If both number of formal study years and education levels were available in the cohort, we classified participants based on years of formal education. For the four cohorts of relatively young European participants (BATS, DCCT, RAINE and WESDR; total n =2,349), almost all of them had completed 12 or more years of schooling. We thus chose to categorize individuals with tertiary or university education as the higher education group in these studies. Sensitivity analysis excluding these four cohorts did not appreciably change our meta-analysis results. Genotyping and imputation Detailed information on the genotyping platforms and QC procedures for each study is provided in Supplementary Table 2 and Supplementary Note 1 . Each study applied stringent QC filters for GWAS. In general, duplicate DNA samples, individuals with low call rate (<95%), gender mismatch or ethnic outliers were excluded. SNPs were excluded if low genotyping call rate (>5% missingness), monomorphic SNPs, with minor allele frequency (MAF) <1% or in Hardy–Weinberg disequilibrium ( P <10 −6 ). After QC filtering, the array genotypes of each study were imputed using the 1000 Genomes Project data as reference panels (build 37, phase 1 release, March 2012) with the software Minimac [57] or IMPUTE2 (ref. 58 ). Approximately six million SNPs that passed imputation quality thresholds (MACH: r 2 >0.5 or IMPUTE info score >0.5) and with MAF ≥5% were eligible for the meta-analysis ( Supplementary Table 2 ). Statistical models For each study, a linear regression model for each genotyped or imputed SNP was constructed with the mean spherical equivalent as the outcome. We assumed an additive genetic model where the number of risk alleles is an ordinal variable (0, 1 and 2) for directly genotyped SNPs or a continuous variable of allele dosage probability ranging from 0 to 2 for imputed SNPs. The primary analytic model included SNP, education and SNP × education interaction term, as well as age and sex as covariates. Additional adjustments for the top principal components of genomic marker variations were performed in individual studies when applicable (that is, when there was evidence of population stratification). We used the following additive genetic model to test for a joint effect of SNP ( β SNP ) and SNP × education interaction ( β SNP × education ) on mean spherical equivalent: where Y is the mean spherical equivalent and education is a dichotomous variable (0=lower education group and 1=higher education group); cov is a set of covariates such as age, sex and first top five principal components when applicable. For family-based studies, the kinship matrix was estimated empirically from the SNP data and included as a random effect in the generalized mixed model [59] . To test an effect of SNP × education interaction, we assessed β SNP × education from equation (1). The linear regression analyses in each study were conducted with Quickes or ProbABEL for the unrelated samples and MixABEL for family-based data. The command ‘robust’ was used in the above software to calculate the robust (‘sandwich’, Huber-White) s.e. of β SNP and β SNP × education , and error covariance of β , to correct the potential inflation of false positive rate for the interaction P -value [60] . In addition, each study also tested the main effect of education on spherical equivalent by adjusting for age and gender using the linear regression model: where the definition of each variable is the same as in equation (1). We performed meta-analysis of the education effects on mean spherical equivalent in Europeans, Asians (Singapore Chinese versus others) and combined data using a fixed-effect model with inverse-variance weighting (R package ‘meta’). GEWIS join meta-analyses We adopted the JMA approach [17] , [61] , to simultaneously test both SNP main effects and SNP × education interactions for spherical equivalent with a fixed-effect model, using SNP and SNP × education regression coefficients ( β SNP and β SNP × education , respectively) and a β ’s covariance matrix from each study. A Wald’s statistic, following a χ 2 -distribution with two degrees of freedom, was used to test the joint significance of the β SNP and β SNP × education . The JMA was performed with METAL [62] , as previously described by Manning et al . [61] . A Cochran’s Q -test was used to assess heterogeneity of the β -coefficients across studies for the SNP and interaction effects. To test for interaction between the SNP and education, we conducted a secondary meta-analysis of the SNP × education interaction effects for spherical equivalent ( β SNP × education , one degree of freedom), with a fixed-effects model using inverse-variance weighting in METAL; this is a traditional meta-analysis to investigate SNP × education interactions per se . Effects and s.e. of the SNP effect on spherical equivalent in the lower education group ( β SNP ) and higher education group ( β SNP + β SNP × education ) were derived from the JMA output [61] . We used the P -value of 5 × 10 −8 as a significant threshold for JMA test. For the SNP and SNP × education effects for the identified top loci, the P -value threshold for significance was set at 0.0055=0.05/9 (9 index SNPs underlying analyses). We performed a meta-regression to explore sources of heterogeneity in our meta-analysis for three loci showing G × E interactions (R package ‘metafor’). Meta-regression included the following study-specific variables as covariates: study sample size, proportion of individuals in the higher education group, average spherical equivalent, education main effects on spherical equivalent (higher education level versus lower), ethnicity (Asian versus European), study design (independent samples versus family-based studies), study year and average age. Meta-regression was also conducted to test the fold changes of the interaction β -coefficients in Asians versus Europeans for the 39 known myopia loci. The study-specific genomic control inflation factors λ gc for the joint test for SNP and interaction terms ranged from 1.009 to 1.125 with an average of 1.019 ( Supplementary Table 2 ), calculated by the ratio of the observed median χ 2 divided by the expected median of the 2df χ 2 -distribution (1.382). Genomic control correction was applied to each individual study [63] . For studies of small sample sizes ( n <500) with λ gc >1.05, we further, before starting the meta-analysis, excluded SNPs showing significant joint P -value <1 × 10 −5 but neither the SNP nor SNP × education effects supported such an association. Quantile–quantile plots showed only modest inflation of the test statistics in the JMA test (Europeans: λ gc =1.081; Asians: λ gc =1.053; Combined: λ gc =1.092; Supplementary Fig. 1 ), similar to previous GEWIS studies with comparable sample sizes [18] , [19] . We excluded a small number of markers in the meta-analysis with P het <0.0001. The λ gc for the SNP × education interaction term in the individual studies ranged from 1.01 to 1.08, indicating little evidence of test statistic inflation on SNP × education effect for each study. Annotation of genetic variants and gene expression in humans The coordinates and variant identifiers are reported on the NCBI B37 (hg19) genome build and annotated using UCSC Genome Browser [64] . We identified variants within each of the LD blocks ( r 2 ≥0.8) in European and Asian populations of the 1000 Genomes Project (100 kb flanking the top SNP at each locus), to apply functional annotations of transcription regulation using HaploReg [65] and Encyclopedia of DNA Elements [66] data. We also generated funcational association and co-expression network using GeneMANIA [67] , to determine whether the disease-related genes identified in this study and previous GWAS [7] , [8] are functionally connected. To assess gene expression in human tissues, we examined the Ocular Tissue Database and the EyeSAGE database [31] , [68] . The estimated gene and exome-level abundances are available online. Normalization of gene expression used the Probe Logarithmic Intensity Error method with genomic control-background correction [31] . Relationships between genotype and cis regulation of gene expression levels ( Supplementary Table 9 ) were assessed using expression quantitative trait locus associations in multiple human tissues from UK samples [34] , as well as gene expression profiles obtained from GTExPortal database [69] . How to cite this article: Fan, Q. et al . Meta-analysis of gene–environment-wide association scans accounting for education level identifies additional loci for refractive error. Nat. Commun. 7:11008 doi: 10.1038/ncomms11008 (2016).